Spin-motive force due to a gyrating magnetic vortex A change of magnetic flux through a circuit induces an electromotive force. By analogy, a recently predicted force that results from the motion of non-uniform spin structures has been termed the spin-motive force. Although recent experiments seem to confirm its presence, a direct signature of the spin-motive force has remained elusive. Here we report the observation of a real-time spin-motive force produced by the gyration of a magnetic vortex core. We find a good agreement between the experimental results, theory and micromagnetic simulations, which taken as a whole provide strong evidence in favour of a spin-motive force. According to theory, motive forces are described by a generalized Faraday law: , where γ , ħ , and e are the Berry phase [1] , Plank's constant divided by 2 π , and the electron's charge, respectively. When γ is the Aharonov–Bohm phase [2] , this expression gives rise the conventional Faraday law. However, including the spin-Berry phase γ s , in the expression gives rise to a spin-motive force (SMF) [3] , [4] , which has an opposite sense for the majority/minority electrons of a ferromagnet. Because of this spin imbalance, this effect can be electrically detected in ferromagnets as an effective electromotive force (EMF) where P is the average spin polarization of conduction electrons. The non-coplanar spin structure is responsible for the spin Berry phase γ s . We note that the SMF signals arising in a single material are driven by an AC magnetic field, in contrast to the spin voltaic effect [5] , [6] , which is realized in a junction system with the circularly polarized light. Recent experiments involving magnetic domain wall propagation, and magnetization reversal of nano-particles embedded in a magnetic tunnel junction have suggested the existence of the SMF [7] , [8] . In these experiments, however, the signals were detected at a point far away from the spin texture, and the measuring time was much longer than the characteristic timescale of the system's spin dynamics. Thus, investigating the dynamical nature of the SMF by directly probing the local spin structure is particularly pertinent given the recent controversy concerning the evidence in favour of the SMF [9] . A magnetic vortex has a core region with a magnetization normal to the plane of the disc ( Fig. 1a–c ) [10] , [11] , forming such a non-coplanar structure. A time dependence of γ s is introduced by the spin dynamics, induced by applying an external in-plane AC magnetic field of frequency f ex close to f r for resonance [12] . When the core passes through the region between the two terminals shown in Fig. 1d , it will induce a SMF that is proportional to the core velocity v (refs 13 , 14 ). More quantitatively, it can be estimated as , where f ex is the driving frequency, R the radius of gyration (that is, ν= 2 π f ex R ) and 2 r c the core diameter. At resonance, f ex ~ f r , the SMF is a maximum, reflecting the maxima of R and v . In this Article, we verify this estimate both by experiment and by micromagnetic simulations. 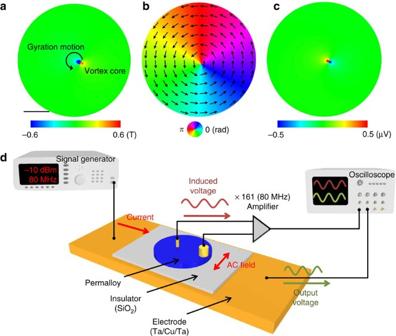Figure 1: Spinmotive force induced by a gyration motion of magnetic vortex and experimental setup. (a–c) Snapshots of perpendicular and in-plane components of magnetization distribution M (a, b respectively) and the corresponding voltage distribution (c) in a ferromagnetic disk obtained by a micromagnetic simulation. The disk contains a magnetic vortex structure. The voltage is due to a spinmotive force generated by the gyrational motion of the vortex core and the corresponding effective electric field is in the direction normal to the core velocity. In the simulation, an external rf magnetic field with amplitudeHrf= 0.5 Oe and the frequencyfex= 80 MHz were used. The diameter of the disk is 4.2 μm. Scale bar corresponds to 1 μm. (d) Measurement setup. A permalloy (Ni80Fe20) disk is put on a coplanar waveguide made of Cu, with an insulating spacer. An rf magnetic field, which induces the core motion, is generated by an electric current applied to the Cu waveguide. The signal was detected using two electrodes deposited on the disk. (e) The overhead view of the device (blue: disk, yellow: pillars). Figure 1: Spinmotive force induced by a gyration motion of magnetic vortex and experimental setup. ( a – c ) Snapshots of perpendicular and in-plane components of magnetization distribution M (a, b respectively) and the corresponding voltage distribution ( c ) in a ferromagnetic disk obtained by a micromagnetic simulation. The disk contains a magnetic vortex structure. The voltage is due to a spinmotive force generated by the gyrational motion of the vortex core and the corresponding effective electric field is in the direction normal to the core velocity. In the simulation, an external rf magnetic field with amplitude H rf = 0.5 Oe and the frequency f ex = 80 MHz were used. The diameter of the disk is 4.2 μm. Scale bar corresponds to 1 μm. ( d ) Measurement setup. A permalloy (Ni 80 Fe 20 ) disk is put on a coplanar waveguide made of Cu, with an insulating spacer. An rf magnetic field, which induces the core motion, is generated by an electric current applied to the Cu waveguide. The signal was detected using two electrodes deposited on the disk. ( e ) The overhead view of the device (blue: disk, yellow: pillars). Full size image Sample structure and measurement setup We prepared devices designed specifically for the observation of the SMF induced by the core gyrational motion. The device structure and the measurement configuration are shown schematically in Fig. 1d . A ferromagnetic micro-disc, 4.2 μm in diameter, is made from a 40nm-thick permalloy (Ni 80 Fe 20 ) film. The aspect ratio is such that a vortex spin structure is formed with its core at the centre of the disc. Below the disc, a copper coplanar waveguide (CWG) is formed, and between the disc and this guide is a SiO 2 electrical insulator layer. Two gold electrode pillars, with different diameters (200 and 600 nm), are asymmetrically placed on the disc to detect the SMF signal. The distance between the smaller pillar A and the centre of the disc is 400 nm. The larger pillar B is placed near the edge of the disc (see Methods ). An AC current with radio frequency (rf) (50–100 MHz) is injected into the CWG by a signal generator. The applied field ( H rf ) is along the in-plane direction to excite the gyrational motion of the core. The induced SMF voltage between the pillars is amplified and measured using a digital oscilloscope (see Methods for details of the measurement). For each measurement, the signal is averaged over more than 60,000 acquisitions. Detection of SMF The resulting signal comprises not only the average of the SMF, but also the conventional EMF induced in the device circuit by the time-varying magnetic flux due to H rf . To extract the SMF signal, the conventional EMF is measured separately for the same disc in the uniform magnetization state obtained by applying a DC external magnetic field (400 Oe) along the in-plane direction (see Methods ) [15] . The periodic SMF obtained by subtracting the EMF has amplitude ~1 μV for an H rf =1.3 Oe with frequency ( f ex ) of 80 MHz, as shown in Fig. 2a . The EMF due to a time-varying magnetic flux, produced by the gyrating vortex, has been numerically calculated and is an order of magnitude smaller than the signal amplitude observed here (see Methods ). 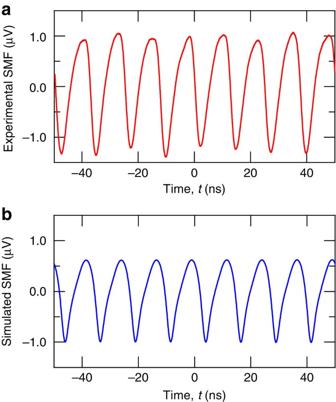Figure 2: Experimental and simulated SMF signals. (a) Experimentally detected spinmotive force as a function of time. The amplitude and frequency of the external (excitation) rf magnetic field isHrf= 1.3 Oe andfex= 80 MHz, respectively. The periodic signal is due to the gyrating vortex core. (b) Simulated time dependence of spinmotive force at the resonance of the gyration motion (80 MHz). The amplitude of the excitation field isHrf= 1.25 Oe. Figure 2: Experimental and simulated SMF signals. ( a ) Experimentally detected spinmotive force as a function of time. The amplitude and frequency of the external (excitation) rf magnetic field is H rf = 1.3 Oe and f ex = 80 MHz, respectively. The periodic signal is due to the gyrating vortex core. ( b ) Simulated time dependence of spinmotive force at the resonance of the gyration motion (80 MHz). The amplitude of the excitation field is H rf = 1.25 Oe. Full size image The experimental results are compared with the SMF calculated in the two-dimensional micromagnetic simulation with parameters appropriate for NiFe. Figure 2b shows the SMF signal simulated for an applied field with amplitude H rf =1.25 Oe and frequency f ex =80 MHz, the latter being close to the resonant frequency ( f r ). The simulated SMF voltage is defined as the difference in the electrochemical potentials between the two electrode pillars placed as in the experiment. The calculated amplitude of ~1 μV is in good agreement with the measured one. Moreover, the shape of the experimental signal, shown in Fig. 2a , with its sharp negative periodic spikes indicating the close approach of the core to the pillar A, is successfully reproduced in the simulation. Excitation frequency dependence of the amplitude of SMF Figure 2a,b displays the raw data. When comparing the frequency dependence of the experimental and simulated amplitudes, it should be borne in mind that the amplifier has a cutoff frequency of about 100 MHz. Namely, the amplitudes and phases of the measured harmonic signals do not reflect those of the original signals. The fundamental signal is determined using a fast Fourier transform filter (see Methods ). The resulting experimental SMF amplitude as a function of frequency f ex of the applied field, for an amplitude H rf =1.0 Oe is shown in Fig. 3a. A peak is seen at about f r (~80 MHz), in good agreement with the experimental f r . The simulated SMF amplitude, for H rf =1.0 Oe ( Fig. 3b ), has a peak at f r (85 MHz). At f r , because the radius R of the core gyration is greatest, the core orbit is closest to the pillar A. 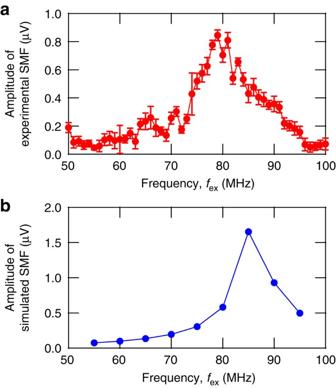Figure 3: Excitation frequency (fex) dependence of the amplitude of the spinmotive force. (a) Experimental result, (b) simulation result forHrf= 1.0 Oe. Figure 3: Excitation frequency ( f ex ) dependence of the amplitude of the spinmotive force. ( a ) Experimental result, ( b ) simulation result for H rf = 1.0 Oe. Full size image Excitation frequency dependence of the amplitude of SMF Finally, we discuss the H rf dependence of the SMF amplitude. 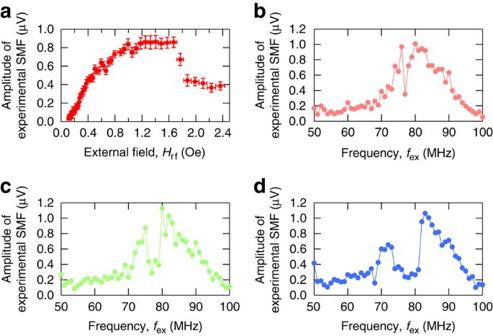Figure 4: Experimental amplitude of spinmotive force. (a) As a function of the rf magnetic field (Hrf) forfex= 80 MHz. (b–d) As a function of excitation frequency (fex) forHrf= 1.3, 1.6, and 2.1 Oe. Figure 4a shows the experimental SMF amplitude as a function of H rf for a fixed f ex =80 MHz. Below ~1.6 Oe, the amplitude increases monotonically with H rf , as expected, because the radius and velocity of the core motion increases. The abrupt drop at ~1.7 Oe is attributed to the onset of random switching of the core polarity [16] . The magnetization in the core is perpendicular to the disc plane and can assume two different directions or polarities (up or down). It is known that when the core velocity exceeds a certain value (~250–300 m s −1 ) [17] , the switching of the polarity becomes more frequent. Theory also predicts, for the current placement of the electrodes relative to the direction of the applied field, that there is no core polarity phase difference of the steady-state signals. (There would be a 90° phase shift if the pillar configuration is rotated by 90° (refs 12 , 18 ).) However, core switching is experimentally known to occur on a timescale that is short compared with the period of oscillations and results in a sudden phase that is shift. The resulting transient should exist for α −1 periods. It follows that when the probability of a reversal approaches unity the signal is strongly suppressed, because our results correspond to an average over ~60,000 acquisitions. Figure 4: Experimental amplitude of spinmotive force. ( a ) As a function of the rf magnetic field ( H rf ) for f ex = 80 MHz. ( b – d ) As a function of excitation frequency ( f ex ) for H rf = 1.3, 1.6, and 2.1 Oe. Full size image The effect of this core reversal can also be seen in the frequency ( f ex ) dependence of the SMF amplitude. The data for H rf =1.3, 1.6 and 2.1 Oe are shown in Fig. 4b–d . Dips are seen at around f r , whereas there was no discernible dip for H rf =1.0 Oe ( Fig. 3a ). For H rf =1.3 Oe, there is a narrow dip just below 80 MHz, implying a frequent core reversal at this field and frequency. The dip becomes wider as H rf is increased to 1.6 Oe and then to 2.1 Oe, which is also consistent with the idea that the critical velocity for core reversal occurring at frequencies further from resonance. In summary, by comparing theoretical, experimental and numerical results, we have demonstrated that a gyrating vortex core produces a spin-motive force in the direction transverse to its motion. In effect, such a non-uniform spin structure can work as a built-in nano-spin–battery, the output of which is tunable by the magnitude and frequency of the external driving field. Compared with the maximum amplitude that one would naively expect for such a motive force, hf ex /e , the observed amplitude is enhanced by a factor proportional to the orbital radius divided by the core diameter. Measurement setup The amplifier has a band-pass characteristic with low- and the high-frequency cutoffs of 1 kHz and 100 MHz, respectively. The amplified output voltage ( V out ) is monitored by an oscilloscope. A high-pass filter with the cutoff frequency of 27.5 MHz was inserted between the amplifier and the oscilloscope to remove the unwanted DC and low-frequency signals. The maximum voltage gain, between the cutoff frequencies, was 46 dB (the voltage gain G v ~200) and G v at 80 MHz was 161. All signals shown here were average of 65,534 acquisitions. Ordinary electromotive force induced by RF field The amplified signal, which includes the ordinary EMF V out for H dc =0 and for H dc =400 Oe are shown in Fig. 5a,b , where H dc is the DC in-plane external magnetic field. A H dc of 400 Oe was confirmed to be strong enough to put the disc in a single-domain state [15] . Fig. 5c shows the difference signal. In Fig. 2a , the amplitude of the difference signal was divided by G v . 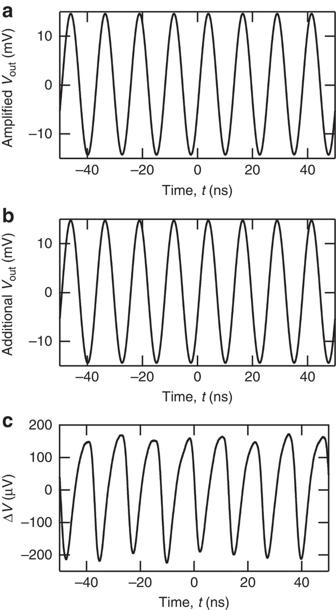Figure 5: The output voltage signals. (a) atHdc= 0 and (b) 400 Oe. (c) The difference signal. Figure 5: The output voltage signals. ( a ) at H dc = 0 and ( b ) 400 Oe. ( c ) The difference signal. Full size image Numerical calculations The numerical calculations are performed as described in ref. 13 . The Landau–Lifshiz–Gilbert equation is solved using the fourth-order Runge–Kutta method. The NiFe disc contains a magnetic vortex structure of 4.2 μm in diameter, and thickness 40 nm. The saturation magnetization was taken to be 4 πM s =1 T, the exchange stiffness A =1×10 11 J m −1 , and the anisotropy constant K =0, and the Gilbert damping coefficient α=0.01. The system is divided into cells of size 5 nm×5 nm×40 nm. The time evolution is determined using 1 ps time steps. Radius of the core motion as a function of excitation frequency is shown in Fig. 6 . 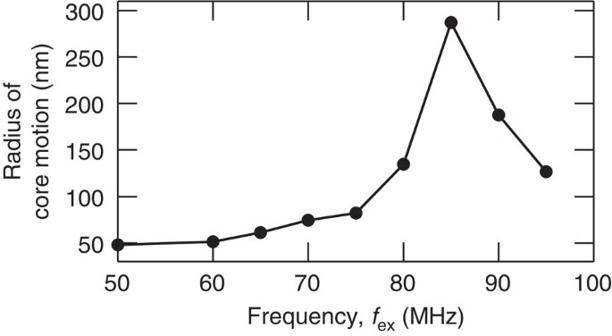Figure 6: Radius of the core motion. As a function of excitation frequency forHrf= 1.0 Oe. Figure 6: Radius of the core motion. As a function of excitation frequency for H rf = 1.0 Oe. Full size image Ordinary electromotive force induced by vortex dynamics The magnitude of the usual EMF produced by the gyrating vortex has been estimated by a numerical calculation of the total time-varying magnetic flux and its time derivative. The geometry is that of the real device. The NiFe disc is divided into cells for the numerical calculation. The total magnetic flux density B was first calculated by integrating the magnetic flux densities induced by each cell. To calculate the total magnetic flux, B is integrated over the area surrounded by the electrodes, which are connected to the pillars, as illustrated in Fig. 7 , On this basis, the EMF due to the vortex motion was estimated to be at most ~100 nV for f ex =80 MHz and H rf =1.0 Oe. 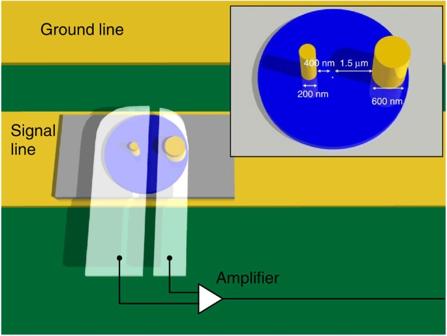Figure 7: Experimental configuration of the electrodes. The magnetic flux is calculated for the configuration, as shown. Figure 7: Experimental configuration of the electrodes. The magnetic flux is calculated for the configuration, as shown. Full size image Fast Fourier transform (FFT) filter First, the FFT of the difference signal is obtained. Then, the spectra below 27.5 MHz and above 100 MHz are removed. Next the amplitude is divided by the frequency-dependent gain of the amplifier and the inverse FFT performed. The resulting amplitudes are shown in Figs 3 and 4 . How to cite this article: Tanabe, K. et al . Spin-motive force due to a gyrating magnetic vortex. Nat. Commun. 3:845 doi: 10.1038/ncomms1824 (2012).